Self-similarity of contact line depinning from textured surfaces The mobility of drops on surfaces is important in many biological and industrial processes, but the phenomena governing their adhesion, which is dictated by the morphology of the three-phase contact line, remain unclear. Here we describe a technique for measuring the dynamic behaviour of the three-phase contact line at micron length scales using environmental scanning electron microscopy. We examine a superhydrophobic surface on which a drop’s adhesion is governed by capillary bridges at the receding contact line. We measure the microscale receding contact angle of each bridge and show that the Gibbs criterion is satisfied at the microscale. We reveal a hitherto unknown self-similar depinning mechanism that shows how some hierarchical textures such as lotus leaves lead to reduced pinning, and counter-intuitively, how some lead to increased pinning. We develop a model to predict adhesion force and experimentally verify the model’s broad applicability on both synthetic and natural textured surfaces. The adhesion of liquid drops to solid substrates, whether it be the ratcheting of drops up a bird’s beak [1] or the anisotropic wetting on butterfly wings [2] and spider silk [3] , is determined by the morphology of the three-phase contact line [4] . Similarly, controlling the mobility of drops and bubbles along surfaces is crucial for many industrial processes, ranging from phase-change heat transfer [5] , [6] , [7] , [8] to biomedical devices [9] , [10] . The dynamic behaviour of the contact line is in turn governed by surface heterogeneities that act as pinning sites to produce local deformations, ultimately leading to contact angle hysteresis and the adhesion of a macroscopic contact line [11] , [12] , [13] , [14] . Recent studies have highlighted the need for a more complete picture of the contact line across multiple length scales [15] , [16] . Despite their importance, dynamic imaging of these microscale deformations has been challenging and particularly elusive in the case of non-wetting drops. Superhydrophobic surfaces utilize a combination of surface chemistry [17] and texture to promote a Cassie–Baxter (CB) wetting state, in which the drop rests atop roughness features forming a composite interface [18] , [19] , [20] , [21] . Adhesion is substantially reduced in the CB state, particularly when multiple length scales are employed [22] , but it is not altogether eliminated. In fact, the adhesion of CB drops represents an almost ideal case of strong dilute defects for investigating the effects of contact line pinning [23] . When a CB drop is moved across a surface, the advancing portion of the contact line simply lies down onto the next roughness features and contributes negligible resistance to drop motion. The deformations due to pinning are localized at the receding region, and as the contact line is displaced, it is hypothesized that micro-capillary bridges are formed at each pinning site [11] , [24] , [25] . For the contact line to move, the micro-capillary bridges must somehow detach from the surface, either by depinning and receding from each roughness feature, or by necking and rupturing. Although the complete mechanism is not known, the global adhesion of the entire liquid drop is dependent on the detachment of these micro-capillary bridges. After numerous studies [24] , [26] , [27] , [28] , [29] , [30] , [31] , [32] , several details of the behaviour of these micro-capillary bridges remain uncertain. Currently, models based on per-pillar adhesion force rely on a correction factor [23] , [33] and computational models rely on satisfying the Gibbs criterion to result in depinning of the capillary bridges [34] . This latter assumption states that as a contact line recedes around a sharp corner, it will remain pinned until it reaches the intrinsic receding angle [35] . This assumption remains to be validated experimentally, as the microscopic receding contact angle of a Cassie droplet on a superhydrophobic surface has not yet been measured. In a study by Chibbaro et al., [36] the authors investigated capillary filling using three computational methods: molecular dynamics, lattice Boltzmann equations and computational fluid dynamics. Surprisingly, they found that for a meniscus advancing over obstacles below a certain size, the Gibbs criterion breaks down due to coalescence of the meniscus with nearby condensed molecules. However, these violations of the Gibbs criterion disappear once the obstacles are made large enough. Therefore, it would be important to also experimentally establish the smallest length scale at which the Gibbs criterion is still satisfied. Experimental investigations of wetting and contact angles at very small length scales are rare. Recently, Mirsaidov et al . [37] used an electron beam to induce movement of drops of water as small as 10–80 nm in diameter and observed unusually-shaped toroidal drops. Although they did not measure nanoscale contact angles directly, the drops nevertheless exhibited advancing and receding fronts as they moved along a surface. There have been only a handful of experimental investigations of micro-capillary bridges, and all high-resolution imaging has been restricted to static drops [24] , [38] , [39] , [40] , [41] , [42] , [43] . Though some have examined the dynamic behaviour, the limited resolution of the three-dimensional details leaves the deformation processes unclear [23] , [33] , [44] , [45] . Furthermore, the effect of multiple length scales on both the behaviour of micro-capillary bridges and macroscopic adhesion of drops remains unresolved. Here we present a method that allows for direct observation of the dynamics of the microscopic contact lines of non-wetting drops to provide quantitative measurements of the deformations at micron length scales. This method allows us to relate the deformations of the contact line to the geometry of the pinning sites. We apply this approach to the specific situation of superhydrophobic surfaces and reveal a self-similar mechanism of contact line depinning. This understanding leads to the prediction of the adhesion force of a drop to a hierarchically textured surface based on the geometry of the roughness features. Dynamic imaging of microscale deformations An environmental scanning electron microscope (ESEM) was used to observe the moving contact line of a water droplet at micron length scales. A 10 μl water drop was affixed to the end of a copper wire, which allowed the drop to be held against a vertically oriented surface and also provided a cooling flux to minimize evaporation ( Fig. 1a ). By rotating the motorized stage of the ESEM, the droplet was swept across the surface at a velocity of 2 μm s −1 while observing the depinning events of the contact line at micron length scales ( Fig. 1b ). The surfaces consisted of silicon micropillars with width w =10 μm, height h =10 μm, edge-to-edge spacing s varying from 3.3 μm to 75 μm. The surfaces were coated with a hydrophobic modifier (tridecafluoro-1,1,2,2, tetrahydrooctyl-trichlorosilane). Advancing and receding contact angles of DI water on a smooth silicon surface treated with the hydrophobic modifier were 120°±2° and 90°±3°, respectively. 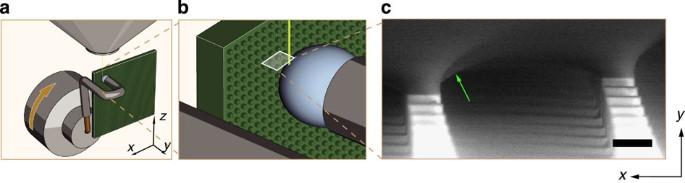Figure 1: ESEM fixture and movie frame. (a) Experimental apparatus within an ESEM chamber. A water droplet is held against a superhydrophobic micropillar surface by a copper wire. The 10 μl drop is cooled by a Peltier device and swept across the surface (xdirection) by rotating the ESEM stage about theyaxis. (b) Illustration of electron beam imaging area with respect to droplet contact line. (c) Single frame from movie of water droplet receding along superhydrophobic micropillars in the positivexdirection shows capillary bridge formation. Arrow indicates penultimate capillary bridge. Scale bar, 10 μm. For complete movie, seeSupplementary Movie 1. Figure 1: ESEM fixture and movie frame. ( a ) Experimental apparatus within an ESEM chamber. A water droplet is held against a superhydrophobic micropillar surface by a copper wire. The 10 μl drop is cooled by a Peltier device and swept across the surface ( x direction) by rotating the ESEM stage about the y axis. ( b ) Illustration of electron beam imaging area with respect to droplet contact line. ( c ) Single frame from movie of water droplet receding along superhydrophobic micropillars in the positive x direction shows capillary bridge formation. Arrow indicates penultimate capillary bridge. Scale bar, 10 μm. For complete movie, see Supplementary Movie 1 . Full size image A single frame from an ESEM movie is shown in Fig. 1c depicting the formation of capillary bridges. Movies of the depinning events on various surfaces are provided in Supplementary Movies 1 , 2 , 3 , 4 . Some important observations can be immediately drawn from the high-resolution images ( Fig. 2 ). It is clear that the macroscopic contact line is not continuous, but is instead composed of a multitude of microscopic contact lines at the top of each pillar. The difference in behaviour between the advancing and receding contact line is apparent in Fig. 2a , in which the advancing contact line lays down onto the next roughness features with a contact angle of ~180° before advancing further. At the receding contact line, numerous micro-contact lines sit at the bases of capillary bridges, which are stretched vertically until they detach from the pillars (see Supplementary Table S1 and Supplementary Note 1 for detailed discussion of bridge detachment). The deformations range from severely distorted capillary bridges sitting on top of micropillars at the periphery of the contact patch to smaller distortions at interior micropillars ( Fig. 1c ). Because the vapour–liquid interface at the centre of the contact patch sags between pillars [46] , [47] , there should be a region over which the vapour–liquid interface is nearly flat, as it begins to deform vertically upwards near the periphery of the contact patch. The extent of the deformation depends on the surface tension of the liquid, and on the density and strength of the pinning features. Lower surface tensions should result in only partially formed peripheral capillary bridges and no interior bridges, as observed recently with cured epoxy drops [41] , [42] . Nevertheless, we observe fully formed peripheral capillary bridges that can be approximated as catenoids atop a sharp-edged disk [48] , [49] . The details of the shape of the multiple catenoids at the base of a spherical drop would be difficult to describe analytically, so we make further simplifying assumptions. We approximate the capillary bridges in the vicinity of the micro-contact lines to have two constant principal radii of curvature, as highlighted in Fig. 3 : r 1 in the plane of the surface, corresponding to the radius of the bridge, r 2 corresponding to the arch between adjacent bridges. The first radius of curvature is constrained by the pinned micro-contact line to be approximately equal to the half-width of a pillar: r 1 ~w/ 2. The second radius of curvature can be calculated by considering the mean curvature of the drop. Neglecting the effects of gravity, the mean curvature of the drop H must remain constant everywhere: H= 2 /R , where R is the radius of the drop. Locally to the capillary bridges, the mean curvature can be estimated by H= 1 /r 1 +1 /r 2 . In the limit that the radius of the drop R >> r 1 , the second radius of curvature between peripheral micropillars can attain a minimum value approximately equal to the half-width of the pillar: r 2 ~w/ 2. The radius of curvature between micropillars close to the centre of the contact patch can be much larger than w /2, and simply scales as the radius of the drop: r 2 ~R (ref. 46 ). Thus, the extent of the deformations around each peripheral capillary bridge scales with the dimensions of the roughness features. This is consistent with previous observations of contact line distortions at larger length scales [14] , [43] . When the micropillars are sparsely spaced ( s >2 w ), the deformations of a capillary bridge will not interact with those of an adjacent capillary bridge ( Fig. 3a ), corresponding to the condition of dilute defects [11] . As the spacing between roughness features decreases, we see that adjacent bridges begin to interact ( Fig. 3b ). This leads to a shorter capillary bridge with a larger contact angle. A similar interaction of menisci has been shown in the case of liquid imbibition through square pillar arrays [50] . 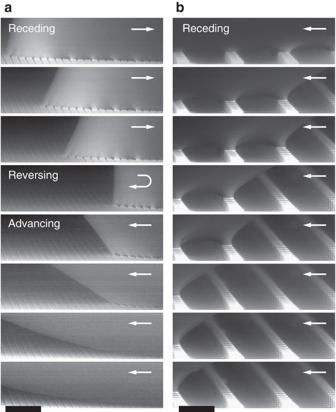Figure 2: Image sequences of moving contact line. (a) Receding and advancing contact line on micropillar array with 3.3 μm spacing. Arrow indicates direction of drop movement. Scale bar, 50 μm. For complete movie, seeSupplementary Movie 2. (b) Receding contact line on micropillar array with 40 μm spacing. Arrow indicates direction of drop movement. Scale bar, 50 μm. For complete movie, seeSupplementary Movie 1. Figure 2: Image sequences of moving contact line. ( a ) Receding and advancing contact line on micropillar array with 3.3 μm spacing. Arrow indicates direction of drop movement. Scale bar, 50 μm. For complete movie, see Supplementary Movie 2 . ( b ) Receding contact line on micropillar array with 40 μm spacing. Arrow indicates direction of drop movement. Scale bar, 50 μm. For complete movie, see Supplementary Movie 1 . 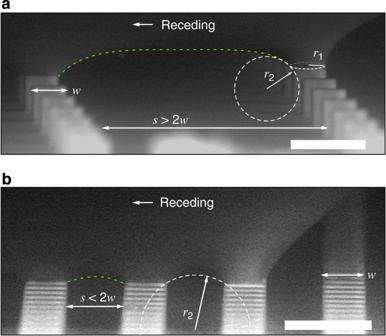Figure 3: Capillary bridge geometry as a function of roughness feature spacing. (a) Representative ESEM frame showing a water drop receding from the right at a velocity of 2 μm s−1on micropillars spaced 75 μm apart, with profile of capillary bridge highlighted; scale bar, 20 μm. (b) Representative ESEM frame showing a water drop receding from the right at a velocity of 2 μm s−1on micropillars spaced 15 μm apart, with profile of capillary bridge highlighted. Scale bar, 20 μm. Full size image Figure 3: Capillary bridge geometry as a function of roughness feature spacing. ( a ) Representative ESEM frame showing a water drop receding from the right at a velocity of 2 μm s −1 on micropillars spaced 75 μm apart, with profile of capillary bridge highlighted; scale bar, 20 μm. ( b ) Representative ESEM frame showing a water drop receding from the right at a velocity of 2 μm s −1 on micropillars spaced 15 μm apart, with profile of capillary bridge highlighted. Scale bar, 20 μm. Full size image Most significantly, we are able to directly measure the microscopic contact angle θ μ at the base of each micro-capillary bridge as shown in Fig. 4 . Our observations show that it can take any value ranging from the advancing contact angle to the intrinsic receding contact angle. The microscopic contact angle reaches a minimum receding value immediately before a capillary bridge detaches from a micropillar: . This microscopic receding contact angle is consistent across all micropillars and is approximately equal to the intrinsic receding angle on a smooth silanized substrate measured using a goniometer: θ r =90°±3°. This observation indicates that the Gibbs criterion for depinning is indeed met at the top surface of the micropillars. In the current study, the microscopic contact angle at the outer edge of a peripheral micropillar is less than that at the interior edges by more than 5° as seen in Fig. 3a , indicating that a capillary bridge will depin from the outer edge of a micropillar as put forth in recent studies [29] , [31] . As the receding angle condition for depinning is always met first on the outer portion of a flat-topped micropillar, the depinning condition is never reached at the interior portion. 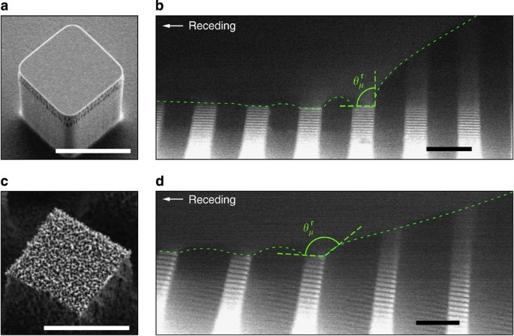Figure 4: SEM micrographs of micro-contact line. (a) SEM micrograph of smooth micropillar. Scale bar, 10 μm. (b) ESEM frame of water droplet receding on smooth micropillars with 15 μm spacing. Microscale receding contact angleθμr=86°±5° (approximately equal to that on a smooth surface:θr=90°±3°). Scale bar, 20 μm. (c) SEM micrograph of nanograss micropillar. Scale bar, 10 μm. (d) ESEM frame of water droplet receding along nanograss-covered micropillars with 25 μm spacing. Microscale receding contact angleθμr=140°±5° (approximately equal to that on a planar nanograss surface:=145°±3°). Scale bar, 20 μm. SeeSupplementary Movie 4. Figure 4: SEM micrographs of micro-contact line. ( a ) SEM micrograph of smooth micropillar. Scale bar, 10 μm. ( b ) ESEM frame of water droplet receding on smooth micropillars with 15 μm spacing. Microscale receding contact angle θ μ r =86°±5° (approximately equal to that on a smooth surface: θ r =90°±3°). Scale bar, 20 μm. ( c ) SEM micrograph of nanograss micropillar. Scale bar, 10 μm. ( d ) ESEM frame of water droplet receding along nanograss-covered micropillars with 25 μm spacing. Microscale receding contact angle θ μ r =140°±5° (approximately equal to that on a planar nanograss surface: =145°±3°). Scale bar, 20 μm. See Supplementary Movie 4 . Full size image Depinning from hierarchical textures We imparted a second roughness scale by etching silicon nanograss [51] into the tops of the micropillars while leaving the dimensions of the first scale unchanged. The contact line of a water drop on these samples was observed with the ESEM in the same manner as before. Figure 4 shows a comparison of the microscale receding contact angle observed on these two types of surfaces measured immediately before detachment of the outer-most capillary bridge. On nanograss-covered micropillars, the microscale receding contact angle increases to and is about equal to the macroscopic receding angle measured using a goniometer on a sample with only a nanograss texture ( ), indicating that the Gibbs criterion is met for each of the two classes of surfaces (smooth micropillars and nanograss-covered micropillars). We observe a higher microscale receding angle for the capillary bridges on the nanograss-covered micropillars as compared with the smooth micropillars. We propose that this is due to a self-similar depinning mechanism, for which the total pinned length of the contact lines at each level of the hierarchical roughness must be taken into account. Considering a droplet sitting on a surface comprising multiple levels of roughness features ( Fig. 5a ), the apparent macroscopic contact line of the drop comprises the zeroth level of hierarchy and will actually be divided into many smaller contact lines, each sitting on top of a roughness feature at the first level ( Fig. 5b ). The receding angle exhibited by the capillary bridges local to the first level of hierarchy will be different from that exhibited by a drop observed at the zeroth level (the macroscopic contact angles measured by a goniometer). The microscale contact angle on smooth micropillars observed by the ESEM is synonymous with . If the contact lines of these first-level capillary bridges are observed at an even smaller length scale, we hypothesize that they will be divided into even smaller contact lines, each sitting on top of a roughness feature at the second level of hierarchy ( Fig. 5c ). The receding angle of these second-level capillary bridges local to the second level of hierarchy will in turn be different from that observed at the first length scale. This self-similar pattern of subdivided contact lines and differing local contact angles may be continued down successive levels until reaching a level n that exhibits a homogeneous wetting interface [25] . At this cutoff level, the contact line on each roughness feature will be continuous. Thus, the actual pinned length of the apparent contact line at any level will be determined by the geometry of the roughness features at all smaller levels, if they exist. If the tops of the roughness features at the cutoff level are also flat, as is the case with the smooth micropillars, the local receding angle should approach the intrinsic receding angle, that is, . 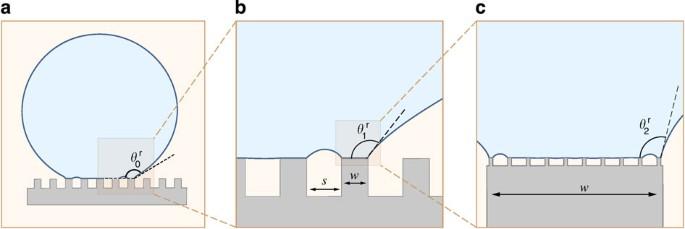Figure 5: Schematic of self-similar contact line pinning. (a) A liquid droplet that rests in a Cassie–Baxter state on a hierarchical surface exhibits an apparent receding angleθ0r. (b) The apparent contact line of the drop is divided into many smaller first-level contact lines, each at the top of a first-level roughness feature with widthwand spacings. Each of these first-level contact lines sits at the base of a first-level capillary bridge, which has a local receding contact angleθ1r. (c) The apparent contact line of each second-level capillary bridge is further divided into smaller second-level contact lines, each atop a second-level roughness feature. Each second-level contact line sits at the base of a second-level capillary bridge, which has a local receding contact angleθ2r. Figure 5: Schematic of self-similar contact line pinning. ( a ) A liquid droplet that rests in a Cassie–Baxter state on a hierarchical surface exhibits an apparent receding angle θ 0 r . ( b ) The apparent contact line of the drop is divided into many smaller first-level contact lines, each at the top of a first-level roughness feature with width w and spacing s . Each of these first-level contact lines sits at the base of a first-level capillary bridge, which has a local receding contact angle θ 1 r . ( c ) The apparent contact line of each second-level capillary bridge is further divided into smaller second-level contact lines, each atop a second-level roughness feature. Each second-level contact line sits at the base of a second-level capillary bridge, which has a local receding contact angle θ 2 r . Full size image The apparent contact line at any level can be projected onto the tops of the roughness features of the next smaller-scale level. The projected contact line will traverse a number of individual roughness elements, as illustrated in Fig. 6a , in which a portion of a projected contact line traverses seven square micropillars. This hypothetical drop will be pinned to both the peripheral micropillars and the interior micropillars, but significant distortion occurs only at the micropillars that sit directly under the projected contact line. The total pinned length is simply the perimeter of each micropillar P multiplied by the number of peripheral micropillars N . The effective pinned fraction φ of a projected contact line of length l can then be found as φ=NP/l . As the number of micropillars per length N/l is equal to the inverse of the average micropillar pitch τ , the pinned fraction can be rewritten as φ = P / τ . Thus, if the roughness features are sparsely spaced, only a small fraction of the projected contact line will be pinned ( Fig. 6b , row 1). However, if the pillars are packed densely, then the pinned fraction will increase. In some cases, φ may be greater than 1, indicating that the sum of the lengths of the contact lines of the peripheral capillary bridges is greater than the length of the projected contact line ( Fig. 6b , row 2). 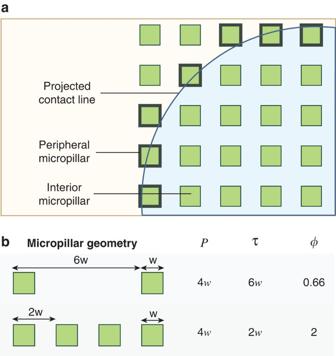Figure 6: Pinned fraction schematics. (a) A contact line projected on a textured surface will be pinned to a number of peripheral micropillars. (b) Effect of texture geometry on pinned fraction. Micropillars with sufficiently dense spacings will result in pinned fractions greater than 1. Figure 6: Pinned fraction schematics. ( a ) A contact line projected on a textured surface will be pinned to a number of peripheral micropillars. ( b ) Effect of texture geometry on pinned fraction. Micropillars with sufficiently dense spacings will result in pinned fractions greater than 1. Full size image The pinned fraction concept can be further applied to structures with multiple hierarchies. Just as the apparent macroscopic contact line of a millimetric drop can be projected onto the tops of the micropillars to obtain the number of peripheral micro-capillary bridges, the contact lines of the micro-capillary bridges can be projected onto the tops of the nanoscale features to find the number of peripheral nano-capillary bridges. The total pinned fraction of a macroscopic contact line at the zeroth level Φ 0 can be calculated for a surface with n hierarchical roughness levels by the product of the pinned fraction at each level: where P i and τ i are the perimeter and average pitch, respectively, of the roughness features at the i th level of the hierarchy. The quantity l 0 Φ 0 then gives the total pinned length of a projected contact line of length l 0 sitting on a surface with n roughness levels. This total pinned length is equal to the sum of the lengths of contact lines of all peripheral capillary bridges at the n th hierarchical level. Similarly, if we wish to find the total pinned length for a subset of levels starting at j < n , we calculate Φ j by evaluating equation (1) from i = j +1 through n : The total pinned length is then given by l j Φ j , where l j is the perimeter of a roughness feature at the j th level. This is useful, for example, in calculating the total pinned length of an individual micro-capillary bridge sitting on a micropillar that itself has additional finer roughness levels. In this case, l j is equal to the perimeter of the micropillar, and is equal to the product of the pinned fractions on the second level and all finer levels. Finally, as the contact line at the n th level is continuous, it is not subdivided any further and the pinned fraction Φ n =1. Surprisingly, equation (1) indicates that adding multiple roughness levels does not necessarily decrease the total pinned fraction. As an example, consider a surface with one roughness scale consisting of sparse micropillars, such that Φ 0 = φ 1 <1. If we impart an additional level consisting of sparse nanograss such that φ 2 <1, then the total pinned fraction becomes Φ 0 = φ 1 φ 2 , which is less than the original pinned fraction. Indeed, for many familiar hierarchical superhydrophobic surfaces such as lotus leaves, there are two roughness scales, and the pinned fraction at both levels is less than one [52] . However, if the nanograss features had been very densely packed such that φ 2 >1, then the total pinned fraction of the dual-level surface would have been greater than that of the single-level micropillar surface: φ 1 φ 2 > φ 1 . This is the case for some nanotube surfaces for which the pinned fraction can be greater than 3, leading to very high droplet adhesion [53] . The adhesion force of a drop to a hierarchical superhydrophobic surface with discrete roughness features can be determined by considering the force due to surface tension acting along the bases of the capillary bridges. By considering a vertical force balance on the drop ( Supplementary Note 2 and Supplementary Fig. S1 ), the adhesion of the entire drop is predominantly dictated by the vertical component of surface tension acting at the peripheral capillary bridges. The force pinning a single capillary bridge at the j th level can be written as , where P j is the perimeter of an individual roughness feature onto which the bridge is pinned, σ is the liquid–vapour surface tension, θ j is the contact angle local to j th level, and d s is a differential length along the perimeter. In the present case, to estimate the maximum adhesion force before detachment, we approximate the contact angle as being uniform around the entire perimeter of the micropillar and equal to the receding angle local to the j th level , so the previous expression simplifies to (see Supplementary Note 3 for discussion of error analysis). If there exist additional roughness levels, the adhesion of the j th -level capillary bridges will be determined by depinning of capillary bridges at the smaller levels. This will in turn affect the value of . Because of the mechanism of self-similar depinning, the adhesion of the entire j th -level bridge will be governed by the detachment of the capillary bridges atop features at the n th level. As the local receding contact angle at this final level, will be approximately equal to the intrinsic receding angle θ r , the vertical force exerted by a single n th -level peripheral capillary bridge due to surface tension will be , where P n is the perimeter of a roughness feature at the n th level, and θ r is the intrinsic receding contact angle. Finally, the vertical adhesion force of the entire drop can be found by summing the forces due to all of the peripheral n th -level capillary bridges: where l 0 is the length of the projected macroscopic contact line. By normalizing the vertical adhesion force predicted by equation (3) to the adhesion force of a drop with an equivalent base radius on a smooth surface, given by ( F / l ) s = σ sin( θ r ), the resulting ratio suggests that Φ 0 can be considered as a multiplier that reflects the strength of the pinning on the textured surface as compared with that on a smooth surface. Therefore, when Φ 0 >1, the adhesion force per unit length of a contact line on a textured surface should be greater than that on a smooth surface, and vice versa. Because of self-similarity, the adhesion force per unit length of a single capillary bridge atop a feature at the j th level is the same as that of a macroscopic drop sitting on a surface consisting of a texture with levels j +1 through n : In other words, the adhesion force per unit length of the microscopic contact line of a micro-capillary bridge on a single nanograssed micropillar is the same as that of a macroscopic drop on a surface with just a nanograss texture. To validate our hypothesis of self-similar depinning, we compared the adhesion force predicted by equation (3) with experimental observations. Using a tensiometer, we measured the force required to pluck a millimetric drop vertically off of two types of surfaces: smooth micropillars and nanograss-covered micropillars ( Fig. 7a ). There is a significant decrease in adhesion to the nanograss-covered micropillars as compared with the smooth micropillars. Additionally, as the spacing ratio s / w increases, the density of micropillars and the adhesion force both decrease. For both the smooth and nanograss-covered micropillars, the pinned line fraction at the first level is given by φ 1 =4 w /( w + s ). In the case of the nanograss-covered micropillars, there is a second roughness level ( n =2) at a nanometre scale with a pinned fraction φ 2 =0.18±0.05 measured from SEM images ( Supplementary Fig. S3 ). 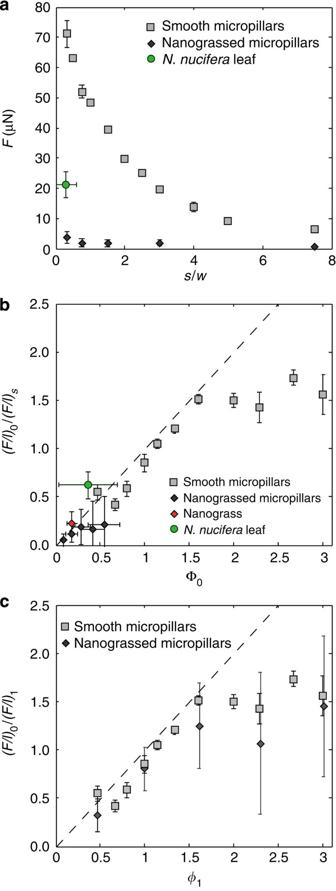Figure 7: Macroscopic adhesion measurements. (a) Adhesion force versus spacing ratio for smooth micropillars, nanograssed micropillars and aN. nuciferaleaf. (b) Ratio of measured adhesion force per unit length of the contact line of a macroscopic drop to that on a smooth surface versus total pinned fraction for smooth micropillars, nanograss micropillars, flat nanograss and aN. nuciferaleaf. Deviation at large pinned fractions is due to interaction of capillary bridges. Dotted line indicates the ratio as predicted by equation (3). Error bars indicate s.e. (c) Adhesion force per unit length of projected contact line of a macroscopic drop normalized to remove the effect of the nanograss hierarchy, plotted against the pinned fraction at the first hierarchy. For the case of nanograssed micropillars, (F/l)0was obtained by measuring the adhesion force of a drop on a nanograss surface and normalizing with the projected length of the contact line. For the case of smooth micropillars, (F/l)0is simply. Dotted line indicates the normalized force as predicted by equation (4). Error bars indicate s.e. Figure 7: Macroscopic adhesion measurements. ( a ) Adhesion force versus spacing ratio for smooth micropillars, nanograssed micropillars and a N. nucifera leaf. ( b ) Ratio of measured adhesion force per unit length of the contact line of a macroscopic drop to that on a smooth surface versus total pinned fraction for smooth micropillars, nanograss micropillars, flat nanograss and a N. nucifera leaf. Deviation at large pinned fractions is due to interaction of capillary bridges. Dotted line indicates the ratio as predicted by equation (3). Error bars indicate s.e. ( c ) Adhesion force per unit length of projected contact line of a macroscopic drop normalized to remove the effect of the nanograss hierarchy, plotted against the pinned fraction at the first hierarchy. For the case of nanograssed micropillars, ( F / l ) 0 was obtained by measuring the adhesion force of a drop on a nanograss surface and normalizing with the projected length of the contact line. For the case of smooth micropillars, ( F / l ) 0 is simply . Dotted line indicates the normalized force as predicted by equation (4). Error bars indicate s.e. Full size image Figure 7b shows ( F / l ) 0 /( F / l ) s — the measured adhesion force per unit projected length of the contact line of a macroscopic droplet normalized to that on a smooth surface—versus the total pinned fraction Φ 0 . For both single- and dual-hierarchy surfaces, and even the lotus leaf, the data collapse onto the line predicted by equation (3). There is a deviation at denser pillar spacings because the roughness features are no longer in the regime of sparse defects, and the peripheral capillary bridges begin to interact with one another. This leads to a larger local receding angle between adjacent pillars as shown in Fig. 3b , thus we would expect the vertical component of surface tension to decrease. Indeed, we find that the normalized adhesion at larger pinned fractions (Φ 0 ≥1.5), which corresponds to the regime of dense spacings, is lower than that predicted by equation (3). The effect of the second level of hierarchy can be factored out by normalizing the measured vertical adhesion force per unit projected length of the contact line of a macroscopic drop from equation (3) with the force per unit length of a capillary bridge on top of the micropillars from equation (4) evaluated at j =1 to obtain the ratio ( F / l ) 0 /( F / l ) 1 . Hence, plotting ( F / l ) 0 /( F / l ) 1 against φ 1 should yield similar results for both smooth micropillars and nanograssed micropillars, as the effect of the texture on top of the micropillars is cancelled. Indeed, Fig. 7c shows that the normalized adhesion forces measured on nanograssed micropillars match well with those measured on smooth micropillars, and as predicted, both lie along a line with a slope of 1. Furthermore, the normalized adhesion forces on the nanograssed micropillars display a similar plateau due to capillary bridges interacting at the microscale level, as seen with the smooth micropillars. However, as the receding angle local to the micropillars is greater for the nanograssed micropillars, they will begin interact at wider spacings than for smooth micropillars and exhibit normalized adhesion forces that are lower than predicted. One might expect that adding any additional level of microtexture to the nanograss would have decreased the adhesion force per unit length. Interestingly, we find that the normalized adhesion of nanograssed micropillars with small s is greater than that of a surface with just a nanograss texture. This can be explained by realizing that the total pinned fraction involves the product of the pinned fractions at both levels, and since φ 1 >1 for s <30 μm, we see how dense nanograssed micropillars ( φ 1 ≥1.5) can exhibit greater normalized adhesion per unit length than a surface with just a nanograss texture. This result is counterintuitive, and shows how additional roughness levels will decrease the adhesion force per length only if the pinned fraction at that level is less than one. As the pinned fraction of a particular level is increased beyond one, that level will act to increase the adhesion force per unit length. However, the adhesion force will saturate when the pinned fraction at that level reaches a critical value ( φ i ≥1.5 in the current case) above which the capillary bridges at that level begin to interact. Using a novel technique for observing the dynamic behaviour of a three-phase contact line and quantitatively measuring contact angles at micron length scales, we show direct evidence that the Gibbs criterion is satisfied at these length scales. We introduce a model that describes a self-similar depinning mechanism and accounts for the effects of the hierarchical roughness features. The model described in equation (4) shows that the adhesion force per unit length of the projected contact line may be either increased or decreased by adding multiple length scales of roughness depending on the pinned fraction of each level of hierarchy. This finding is important for designing surfaces with minimal adhesion, as it quantifies the effect of multiple length scales on the adhesion of a liquid drop on a textured surface: to reduce adhesion, the product of the pinned fractions at all length scales must be less than one. Furthermore, two micropillar geometries that have identical area fractions may have different pinned fractions depending on their perimeter and spacing, whereas any attempt to calculate pinning or hysteresis based on area fraction would yield identical results for the two surfaces. In agreement with our mechanism, experiments have shown that the hysteresis differs depending on the micropillar perimeter and tip geometry [24] , [40] , [53] . Our technique could also enable the detailed imaging of contact line behaviour on complex pillar geometries and on intricate biological surfaces, such as water strider legs [54] and fibre arrays [55] . Fabrication of superhydrophobic substrates. Silicon substrates (n-type ‹100›) were patterned with arrays of square micropillars 10 μm high and 10 μm wide, with spacings ranging from 3.3–75 μm, using standard positive photolithography techniques and deep reactive-ion etching. By performing a plasma etch with O 2 and SF 6 , a silicon nanograss texture was etched into the top surfaces of the micropillar structures. All surfaces were coated with a hydrophobic modifier (tridecafluoro-1,1,2,2, tetrahydrooctyl-trichlorosilane). Advancing and receding contact angles of DI water on a smooth silicon surface treated with the hydrophobic modifier were measured with a goniometer (Model 500, ramé-hart) at 25 °C to be 120°±2° and 90°±3°, respectively. Lotus leaves were generously provided by Marilyn Eigsti of Wonderful Water Lilies, Sarasota, FL. In-situ imaging using ESEM apparatus A Zeiss EVO-55 ESEM was used for imaging. A custom fixture was fabricated to mount the samples vertically in the ESEM and provide cooling with a Deben Coolstage Mk II Peltier cooling stage. A 10 μl water drop was affixed to the end of a copper wire that allowed the drop to be held against a vertically oriented surface, and also provided a cooling flux to minimize evaporation. By rotating the motorized stage of the ESEM, the droplet was swept across the surface at a velocity of 2 μm s −1 while observing the depinning events of the contact line at micron length scales. The chamber of the ESEM was maintained at a pressure of 1,000 Pa. Nanograss pinned fraction High-resolution SEMs were used to estimate the pinned fraction of the silicon nanograss. The perimeters of the tops of the roughness features were identified and measured manually, as well as the distances between adjacent roughness features. A representative frame is shown in Supplementary Fig. S2 . The pinned fraction was taken as the average of the perimeters of the roughness features divided by the average distance between the centroid of each feature. A pinned fraction of 0.18±0.05 was determined as the average value from five SEM images taken at different locations. Macroscale tensiometer adhesion measurements A Sigma KSV 700 tensiometer was used to measure the adhesion force of water drops on superhydrophobic surfaces ( Supplementary Fig. S3 ). A 3 μl drop was held at the end of the force balance and lowered onto a test surface at 0.5 mm min −1 until a compressive force of 1 nN was measured, indicating contact with the surface. The drop was then lifted at 0.5 mm min −1 until detachment, at which point the tensile force and contact patch radius were measured. Measurements were repeated at five locations on each sample. How to cite this article: Paxson, A.T. and Varanasi, K.K. Self-Similarity of contact line depinning from textured surfaces. Nat. Commun. 4:1492 doi: 10.1038/ncomms2482 (2013).